Waveforms for optimal sub-keV high-order harmonics with synthesized two- or three-colour laser fields High-order harmonics extending to the X-ray region generated in a gas medium by intense lasers offer the potential for providing tabletop broadband light sources but so far are limited by their low conversion efficiency. Here we show that harmonics can be enhanced by one to two orders of magnitude without an increase in the total laser power if the laser’s waveform is optimized by synthesizing two- or three-colour fields. The harmonics thus generated are also favourably phase-matched so that radiation is efficiently built up in the gas medium. Our results, combined with the emerging intense high-repetition MHz lasers, promise to increase harmonic yields by several orders to make harmonics feasible in the near future as general bright tabletop light sources, including intense attosecond pulses. The bright, spatially coherent radiation emitted by a laser can be found in numerous research applications, such as spectroscopy, photochemistry, communications, imaging and material processing. Because different applications often demand light in specific spectral regions, large facilities have been built that generate powerful broadband tunable light like synchrotron radiation and free-electron laser. However, for such lights to become widely available, it is desirable that they exist as a tabletop equipment in individual laboratories. From nonlinear optics, it has been well known for years that laser light can be converted from one wavelength to another. In particular, coupling of a laser with an optical waveguide can generate a broadband supercontinuum [1] spanning several octaves, whereas the nonlinear interaction of infrared lasers with gas media can generate high-order harmonics extending to soft and hard X-rays [2] . High-order harmonic generation (HHG) in the X-ray regime represents nonlinear optics at the extreme. When amplified in intensity, HHG can offer valuable tabletop broadband light sources. These light pulses, which can be shorter than subfemtoseconds, can be used to probe the structure and dynamics of atoms, molecules and materials with unprecedented spatial and temporal resolution. High-order harmonic generation is a universal response of atoms and molecules when they are exposed to strong femtosecond laser fields. The highest energy of HHG photon emitted from a single atom is given by ħω c = I p +3.17 U P , where U P is the quiver energy of a free electron in the laser field, I p is the ionization energy of the atom and ħ is the reduced Planck’s constant. With widely available Ti:sapphire lasers operating at a 0.8-μm wavelength, the HHG light has been limited to the extreme ultraviolet (~100 eV). However, for a laser with intensity I L and wavelength λ L , . Thus, with mid-infrared lasers of wavelengths of a few microns, the cutoff energy ħω c can now easily reach the X-ray region [2] . Today the main limitation that prevents HHG from emerging as a useful light source is its low conversion efficiency [3] . Most efforts to enhance HHG yields with single-colour sinusoidal waves have been directed at creating favourable phase-matching conditions in the nonlinear gas medium to efficiently build up macroscopic high harmonics [4] , [5] , [6] . Alternatively, enhancement of HHG can be achieved by two-colour phase control, as first shown experimentally by Watanabe et al. [7] in 1994. Since then many such measurements have been reported ( Supplementary Discussion ) using the fundamental 800-nm laser with its second or third harmonic where the phase between the two colours is locked but can be tuned. Similarly, enhancement of HHG has been predicted in many theoretical simulations ( Supplementary Discussion ). More recently, advancement in optical parametric amplification (OPA) and optical parametric chirped-pulse amplification (OPCPA) technology has made it possible to perform coherent wavelength multiplexing of ultra-broadband (over two or more octaves) pulses with full phase and amplitude control, thus allowing the generation of any optical waveform [8] , [9] , [10] , [11] , [12] , [13] , [14] , [15] , [16] , [17] , [18] . With so many ‘knobs’ accessible, it is of critical importance to develop a general algorithm for optimal waveform control for the efficient enhancement of high-harmonic generation and for other strong field phenomena. In this work, we address how to enhance HHG yields by one to two orders by modifying the waveform of the laser to increase the harmonics from each atom that are favourable for phase-matching. This is accomplished by synthesizing ‘only’ two- or three-colour laser fields without increasing the total laser power. We remark that in an early study [19] a ‘perfect wave’ was derived that can be synthesized with five-colour fields. In comparison, our optimized waveform generates higher harmonic cutoff than the ‘perfect wave’ ( Supplementary Fig. 1 and Supplementary Discussion ) and is synthesized with only a two-colour field. Principle of waveform synthesis High-order harmonics are generated from an atom within each optical cycle. The generation of harmonics can be described by a three-step model [20] , [21] : a bound electron first tunnel-ionizes into the continuum; then it is accelerated by the laser field; and finally it recombines with the parent ion on reversal of the laser field, emitting a high-energy photon. For each returning electron that leads to photon emission, there are two trajectories, called the long and short, depending on the excursion time. Harmonics from the recombination of long-trajectory electrons accumulate large phases. These harmonics are hard to phase-match, and they usually do not contribute to the macroscopic HHG spectra. Therefore, the strategies for modifying the waveform for optimal macroscopic HHG are, first, to increase the laser’s electric fields at ionization times to release more electrons that are needed for the HHG and, second, to enhance short-trajectory electrons over long-trajectory ones. The optimization should be carried out under the constraint that the total ionization be less than 2–5%, to avoid electron plasma in the gas medium that would defocus the laser beam [2] . Another requirement is that the total energy of the laser must not be greatly increased. 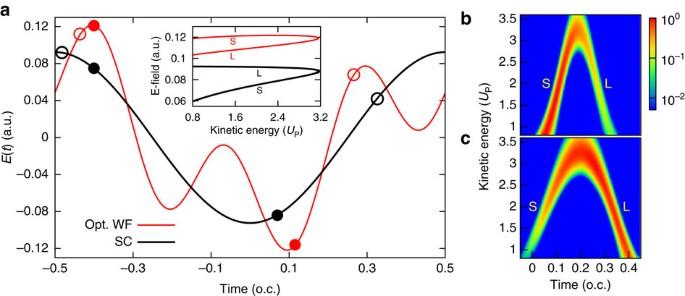Figure 1: Principle of waveform synthesis for optimal high-harmonic generation. (a) Comparison of the electric fields over one optical cycle of the fundamental for a single-colour (SC) sinusoidal wave and an optimally synthesized two-colour field. The optimized waveform (Opt. WF) is synthesized from a fundamental and its third harmonic. The amplitude and phase of each colour field are chosen such that harmonics generated from the synthesized wave are optimized with two constraints: (1) the emissions are dominated by the recombination of the so-called short-trajectory electrons; (2) the total ionization fraction is restricted to below 2–5%. These two constraints guarantee that harmonics generated from each atom in the gas media are favourably phase-matched. On the waveform curves, shown in open and filled circles, are the times when an electron is tunnel-ionized and when it recombines to emit a photon, for an electron that returns with kinetic energy of 2UP. HereUPis defined in terms of the single-colour sinusoidal wave. The open circles are for long-trajectory electrons that have longer excursion time, and the filled circles are for short-trajectory electrons that have smaller excursion time. The inset depicts the electric fields at ionization time versus the kinetic energies of the returning electrons for short- and long-trajectory electrons. For the optimized wave, the field strengths at the ionization times are higher than the single-colour sinusoidal wave, and the fields for the short-trajectory electrons are higher than the long ones. (b) The yields of harmonics emitted from the short- and long-trajectory returning electrons versus the recombination times for the optimized wave, from time-frequency wavelet analysis of the calculated harmonics. (c) Same asbbut for the single-colour wave. Figure 1a depicts two waveforms over one optical cycle: the single-colour sinusoidal wave of the fundamental (black) and the waveform optimized from synthesized two-colour fields (red). For an electron returning with a kinetic energy of 2 U P , the ionization time and the recombination time for the long- (open circles) and short-trajectory electrons (solid circles) are indicated for each waveform. The inset gives the electric fields at ionization times versus the returning electron energies. Comparing the two waveforms, it is clear that the optimized one has higher electric fields at ionization times that lead to more returning electrons, and there are more short-trajectory electrons than long ones. Figure 1b,c show the time-frequency wavelet analysis of HHG calculated using quantitative rescattering theory [22] , [23] ; see Supplementary Methods for the quantitative rescattering theory and the discussion of its validity. The strong enhancement of short-trajectory electrons (labelled ‘S’ in the figure) and the smaller attochirp (steeper slope) [24] for the optimized wave is clearly seen. In the simulation, the wavelength of the fundamental was 1,600 nm and the wavelength of the secondary laser was 533 nm. The target was Ne. For the 1,600 nm alone, we chose an intensity of 3 × 10 14 W cm −2 . The carrier-envelope phase of the fundamental was set at ϕ 1 =0. The optimization returned the peak intensity for the fundamental as 1.98 × 10 14 W cm −2 and 1.32 × 10 14 W cm −2 for the secondary laser, which had the optimized phase ϕ 2 =1.36π. Optimization was performed such that the cutoff and total laser power for the single-colour wave and the optimized wave were about the same. The details of the optimization are given in the Supplementary Information ; see Supplementary Figs 2–9 for two-colour optimization, Supplementary Figs 10–12 for three-colour optimization, Supplementary Methods and Supplementary Discussion . Laser parameters of waveforms obtained from the optimization are given in Supplementary Tables 1–11 . We comment that optimization of harmonics only from short-trajectory electrons was not considered in the previous study [19] . Figure 1: Principle of waveform synthesis for optimal high-harmonic generation. ( a ) Comparison of the electric fields over one optical cycle of the fundamental for a single-colour (SC) sinusoidal wave and an optimally synthesized two-colour field. The optimized waveform (Opt. WF) is synthesized from a fundamental and its third harmonic. The amplitude and phase of each colour field are chosen such that harmonics generated from the synthesized wave are optimized with two constraints: (1) the emissions are dominated by the recombination of the so-called short-trajectory electrons; (2) the total ionization fraction is restricted to below 2–5%. These two constraints guarantee that harmonics generated from each atom in the gas media are favourably phase-matched. On the waveform curves, shown in open and filled circles, are the times when an electron is tunnel-ionized and when it recombines to emit a photon, for an electron that returns with kinetic energy of 2 U P . Here U P is defined in terms of the single-colour sinusoidal wave. The open circles are for long-trajectory electrons that have longer excursion time, and the filled circles are for short-trajectory electrons that have smaller excursion time. The inset depicts the electric fields at ionization time versus the kinetic energies of the returning electrons for short- and long-trajectory electrons. For the optimized wave, the field strengths at the ionization times are higher than the single-colour sinusoidal wave, and the fields for the short-trajectory electrons are higher than the long ones. ( b ) The yields of harmonics emitted from the short- and long-trajectory returning electrons versus the recombination times for the optimized wave, from time-frequency wavelet analysis of the calculated harmonics. ( c ) Same as b but for the single-colour wave. Full size image Two-colour synthesized waveforms To confirm that the one-cycle result in Fig. 1 applies to realistic laser pulses, we synthesize a three-cycle (16 fs of full width at half maximum), 1,600 nm mid-infrared pulse and a visible 533 nm pulse with the same duration, each with a Gaussian envelope. With the optimized pulse, we calculated the HHG spectra generated from a single Ne atom, see Fig. 2a . We observed an enhancement of about two orders in the optimized waveform over the single-colour case. In Fig. 2b we show the HHG spectra after macroscopic propagation in the gas medium. The HHG yields near the cutoff (at about 250 eV) from the optimized waveform maintain two orders of enhancement, but at lower photon energies near 100 eV the enhancement is about three orders. The additional enhancement reflects that there are more short-trajectory electrons contributing to HHG for the optimized wave. Time-frequency wavelet analysis of the harmonic spectra is shown in Fig. 2c–f . Clearly, at the single-atom level the optimized pulse has much stronger contributions from short-trajectory electrons ( Fig. 2c ). After propagation, all the long-trajectory contributions vanish ( Fig. 2d ). In the single-colour case, at the single-atom level the long-trajectory electrons dominate ( Fig. 2e ); after propagation, the short-trajectory electrons dominate, except for a small long-trajectory contribution for low-energy electrons close to U P ( Fig. 2f ). This example demonstrates the importance of optimizing harmonics from short-trajectory electrons, not from both long- and short-trajectory electrons that coexist in the total single-atom harmonics. Inspections of Fig. 2c,e also show that multiple returns (the low-energy ‘bursts’ inside the bigger high-energy ‘bursts’ from the single returns) are much weaker for the optimized wave. 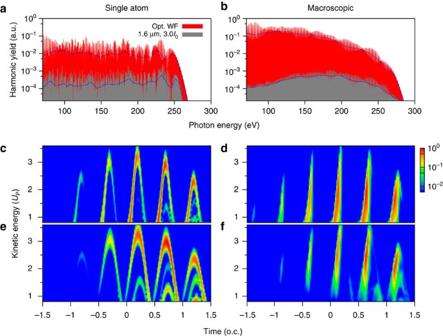Figure 2: Harmonic generation by a sinusoidal and an optimized two-colour fields. The fundamental pulse is a three-cycle (duration is 16 fs), 1,600 nm pulse. The secondary pulse is its third harmonic. For the single-colour wave, the peak intensity is taken at 3.0I0(I0=1014W cm−2). The laser parameters of the two colours for the optimized wave are given in the text. The total pulse energy for the synthesized wave is 10% higher than the single-colour pulse. (a) Single-atom harmonic yields for the two waves, showing that the optimized wave is about two orders stronger than the single-colour one. (b) The yields of high harmonics after macroscopic propagation. In the simulation, the lasers with beam waist of 40 μm are focused 2.5 mm before a 1-mm long gas jet. The gas pressure is 10 Torr. Blue curves inaandbshow the smoothed spectra. (c) Time-frequency analysis of the bursts of harmonics generated by the optimized wave at the single-atom level, showing short-trajectory electrons dominate over long-trajectory electrons. The weak signals (features inside each ‘burst’) at lower kinetic energies are contributions from multiple returns. (d) Time-frequency analysis of the bursts of harmonics after propagation in the gas medium for the optimized wave. All the harmonics from long-trajectory electrons and from multiple returns disappear. This figure illustrates that enhancing short-trajectory electrons from each single-atom response is essential for optimizing the yields of macroscopic harmonics. (e) Single-atom harmonics generated using a single-colour sinusoidal wave, showing strong signals from long-trajectory electrons and from multiple returns (features inside each ‘burst’). (f) Propagated harmonics generated using single-colour sinusoidal waves. This figure shows that most of the harmonics from long-trajectory electrons and multiple returns do not survive phase-matching. Only harmonics from short-trajectory electrons are phase-matched. (o.c. stands for optical cycle of a 1600-nm laser.) Figure 2: Harmonic generation by a sinusoidal and an optimized two-colour fields. The fundamental pulse is a three-cycle (duration is 16 fs), 1,600 nm pulse. The secondary pulse is its third harmonic. For the single-colour wave, the peak intensity is taken at 3.0 I 0 ( I 0 =10 14 W cm −2 ). The laser parameters of the two colours for the optimized wave are given in the text. The total pulse energy for the synthesized wave is 10% higher than the single-colour pulse. ( a ) Single-atom harmonic yields for the two waves, showing that the optimized wave is about two orders stronger than the single-colour one. ( b ) The yields of high harmonics after macroscopic propagation. In the simulation, the lasers with beam waist of 40 μm are focused 2.5 mm before a 1-mm long gas jet. The gas pressure is 10 Torr. Blue curves in a and b show the smoothed spectra. ( c ) Time-frequency analysis of the bursts of harmonics generated by the optimized wave at the single-atom level, showing short-trajectory electrons dominate over long-trajectory electrons. The weak signals (features inside each ‘burst’) at lower kinetic energies are contributions from multiple returns. ( d ) Time-frequency analysis of the bursts of harmonics after propagation in the gas medium for the optimized wave. All the harmonics from long-trajectory electrons and from multiple returns disappear. This figure illustrates that enhancing short-trajectory electrons from each single-atom response is essential for optimizing the yields of macroscopic harmonics. ( e ) Single-atom harmonics generated using a single-colour sinusoidal wave, showing strong signals from long-trajectory electrons and from multiple returns (features inside each ‘burst’). ( f ) Propagated harmonics generated using single-colour sinusoidal waves. This figure shows that most of the harmonics from long-trajectory electrons and multiple returns do not survive phase-matching. Only harmonics from short-trajectory electrons are phase-matched. (o.c. stands for optical cycle of a 1600-nm laser.) Full size image Three-colour synthesized waveforms Can HHG yields be substantially further enhanced by synthesizing three sinusoidal waves instead of only two? With the same simulation method, we searched the optimized waveforms from three pulses with wavelengths of 1,600, 800 and 533 nm. The top three sets of laser parameters obtained from optimization ( Supplementary Table 1 ) resulted in nearly identical waveforms (see Fig. 3a ) and they generated more or less identical HHG spectra, as seen in Fig. 3b . The single-atom HHG yields from this three-colour synthesized waveform are only about two times higher than the yields from the two-colour synthesized waveform examined in Fig. 2 (not shown). For the optimized wave (Index=1 in Supplementary Table 1 ) in the three-colour case, the electric fields at the ionization times (inset of Fig. 3a ) are larger for the long-trajectory than for the short-trajectory electrons. In this example, the prediction from the simple classical three-step model is incorrect. That model fails to include quantum diffusion of electrons between ionization and recombination. The diffusion effect is roughly inversely proportional to the third power of the excursion time, thus reducing more yields for long-trajectory electrons than for short-trajectory electrons [25] . Time-frequency analysis of the calculated HHG, which includes quantum diffusion, indeed indicates that short-trajectory electrons dominate the harmonic yields ( Fig. 3c ) for the optimized wave. 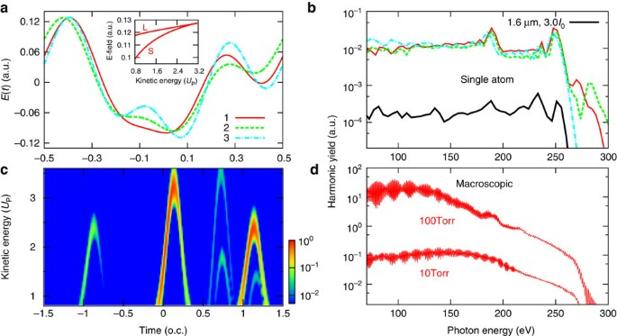Figure 3: Harmonic spectra from three-colour optimized waveforms. The two secondary colours are the second and third harmonics of the fundamental wave, which is 1,600 nm. (a) The waveforms of the top three optimized pulses (laser parameters for Index=1, 2 and 3 are given inSupplementary Table 1). All three waveforms have comparable electric fields near the ionization times (close to −0.4 optical cycles in the figure). The inset shows the electric fields at ionization times for long- and short-trajectory electrons calculated using classical theory (for Index=1 inSupplementary Table 1). (b) Single-atom harmonic spectra (smoothed by using the Bezier curve) for the three top optimized pulses showing nearly identical yields. All of them are two orders stronger than the single colour one. The peak intensity for the single-colour laser is 3.0I0(I0=1014W cm−2). The total peak intensity for the optimized wave is about 3.5I0. The harmonic spectra were generated for a three-cycle pulse (16 fs) for the fundamental wave. The same pulse durations are used for the two other waves. (c) Time-frequency analysis of the harmonic emission, showing one emission per optical cycle of the fundamental wave. The second emission within each cycle is much weaker. This is expected since the waveform shown inaindicates that the peak field in the second half optical cycle is 20–30% weaker compared with the peak field in the first half optical cycle. (d) Macroscopic HHG spectra at two gas pressures of 10 and 100 Torr, respectively. The harmonics beyond 210 eV are continuous that is good for generating isolated attosecond pulses. Figure 3: Harmonic spectra from three-colour optimized waveforms. The two secondary colours are the second and third harmonics of the fundamental wave, which is 1,600 nm. ( a ) The waveforms of the top three optimized pulses (laser parameters for Index=1, 2 and 3 are given in Supplementary Table 1 ). All three waveforms have comparable electric fields near the ionization times (close to −0.4 optical cycles in the figure). The inset shows the electric fields at ionization times for long- and short-trajectory electrons calculated using classical theory (for Index=1 in Supplementary Table 1 ). ( b ) Single-atom harmonic spectra (smoothed by using the Bezier curve) for the three top optimized pulses showing nearly identical yields. All of them are two orders stronger than the single colour one. The peak intensity for the single-colour laser is 3.0 I 0 ( I 0 =10 14 W cm −2 ). The total peak intensity for the optimized wave is about 3.5 I 0 . The harmonic spectra were generated for a three-cycle pulse (16 fs) for the fundamental wave. The same pulse durations are used for the two other waves. ( c ) Time-frequency analysis of the harmonic emission, showing one emission per optical cycle of the fundamental wave. The second emission within each cycle is much weaker. This is expected since the waveform shown in a indicates that the peak field in the second half optical cycle is 20–30% weaker compared with the peak field in the first half optical cycle. ( d ) Macroscopic HHG spectra at two gas pressures of 10 and 100 Torr, respectively. The harmonics beyond 210 eV are continuous that is good for generating isolated attosecond pulses. Full size image One important consequence of three-colour synthesis is that, in each cycle, the optimized waveform generates only one high energy harmonic burst, since the peak electric field of this waveform in the second half cycle (see Fig. 3a ) is 20–30% weaker than the peak field in the first half cycle. Figure 3c shows a single dominant burst of harmonic emission near the centre of the pulse. The harmonics after propagation in the gas medium are shown in Fig. 3d , at two gas pressures. For energies above 210 eV until the cutoff near 250 eV, a continuum spectrum appears that can support an isolated attosecond pulse with central energy at around 230 eV. Figure 3d also shows that higher harmonics at the higher pressure of 100 Torr drop faster than that for the 10 Torr. This is caused by plasma defocusing since electron density in the medium increases with gas pressure. (For other examples of synthesizing three commensurate lasers, see Supplementary Fig. 10 and Supplementary Discussion .) Waveform synthesis in the laboratory The optimization of a waveform by synthesizing two- or three-colour fields usually returns with a few sets of laser parameters that give comparable enhancement of HHG, more so for three- than for two-colour fields (see Supplementary Tables 1 and 2 ). For enhancing HHG, any one of these sets of laser parameters can be implemented in the laboratory. For two-colour synthesis, we observed that the wavelength of the second colour has to be close to the third harmonic of the fundamental. If the second harmonic is used as the second colour, the HHG enhancement is only about 10 times instead of 100 times stronger ( Supplementary Fig. 6 ). The wavelengths of fundamental and secondary waves in the synthesis do not have to be commensurate, nor do their bandwidths have to overlap. For commensurate wavelengths, say, for three colours, the synthesized wave repeats with a new optical period T , which is the lowest integer multiple of the periods of all the three waves. Optimization of waveform synthesis can then be carried out only within this optical cycle T . If the wavelengths are incommensurate, optimization has to be carried out for the whole duration of the wave. In some laboratories, the wavelengths of the wave fields to be synthesized are already fixed in their set-up. Clearly changing the wavelengths in the experiment is harder than changing the intensity and phase of each wave. In Supplementary Information, we have performed optimization for lasers reported in Huang et al. [14] ( Supplementary Fig. 9 ) and Wirth et al. [15] ( Supplementary Figs 11 and 12 where the generation of an isolated attosecond pulse is discussed) with fixed wavelengths. Enhancement of HHG by two orders is obtained if the waveforms in these experiments had been optimized. For each set of optimized laser parameters, small variations in intensity of each wave have only small effects on the enhanced HHG. However, the synthesized waveform depends critically on the relative phases among the input waves. Simulation indicates that if the relative phase deviates by more than 0.2 π from the optimized value, the HHG yield begins to drop substantially ( Supplementary Fig. 3 ). In present-day laser technology, the jitter of the carrier-envelope phase is about 0.1 π under good conditions. Additional jitter may come from the time delay between the pulses. Phase stability of each wave in the synthesis will be the most important controlling factor in the experimental realization of waveform optimization. The optimized waveforms reported here are for optimization of HHG with the constraint that the cutoff is not extended beyond the limit set by the fundamental laser. If different criteria are chosen for the fitness functions in the optimization, different waveforms will be generated. For example, a very different optimized waveform is obtained if long-trajectory electrons are to be enhanced ( Supplementary Fig. 8 ). The present optimization algorithm is easily extended to include other criteria as well as constraints in the simulation. When the synthesis with more colours or direct manipulation of component phases of a supercontinuum [26] becomes practical, it would be interesting to investigate whether further waveform control can significantly enhance the HHG. Finally, to generate usable lights with HHG the effect of phase matching of the harmonics in the gas medium has to be further studied. In a focused laser beam, the peak intensity of the pulse varies in space, thus only the waveform near the laser focus is optimized. In the Supplementary Information, we have carried out a number of simulations to show that enhancement of macroscopic HHG for an optimized wave versus the single-colour one is equal to or higher than that at the single-atom level ( Supplementary Fig. 13 ). However, a more efficient optimization of phase-matching is best done experimentally at individual laboratories. With single-colour mid-infrared lasers, experiments have shown that significant enhancement can be reached if the harmonics are generated in a high-pressure capillary [2] . By optimizing the gas pressure independently, harmonics generated from a 2.0-μm laser versus from a 0.8-μm one have been observed to increase by an order, as compared with harmonics generated with the same pressure [27] . Unless proven otherwise, there is good reason to believe that such additional enhancement can also be accomplished by the synthesized waves with mid-infrared lasers. Waveform synthesis using two- or three-colour fields provides efficient modification of the electric field that enhances harmonic yields from each atom by one to two orders (the factor is larger for smaller total laser power) without much increase in the total laser power. This result has an immediate impact on three research areas in strong field physics. First, applications of mid-infrared lasers for HHG from polyatomic molecules have always been plagued by weak signals, such that data were taken near saturation intensities [28] , [29] where excessive ionization in the medium will reshape the spectra. With waveform-optimized lasers, HHG data can be taken at lower intensities such that the experimental HHG spectra can be used to extract the target structure of a polyatomic molecule directly. Similarly, waveform-optimized lasers also can help laser-induced electron diffraction experiments where the signal is proportional to the flux of laser-driven returning electrons [30] . Laser-induced electron diffraction offers potential for probing molecules with femtosecond temporal and sub-Angstrom spatial resolution. Second, the one- to two-order enhancement of HHG yields from waveform-optimized mid-infrared lasers, if implemented with the emerging intense high-repetition MHz lasers [31] , will increase photon yields per second from what is available today by several orders, thus making it possible to generate usable broadband tabletop light sources in the laboratory. Since the optimized waves also readily generate supercontinuum spectra, intense isolated attosecond pulses are also generated after spectral filtering. Such isolated attosecond pulses, covering photon energies from the extreme ultraviolet to X-rays, can find many applications for probing electron dynamics of atoms, molecules and condensed materials. Finally, waveform-optimized lasers are expected to have great impact on any intense laser-driven processes, including THz generation [32] , laser-plasma interactions [33] and particle acceleration. Clearly, progress in waveform synthesis and optimization will have far-reaching effects on all aspects of strong field physics in the coming years. How to cite this article: Jin, C. et al. Waveforms for optimal sub-keV high-order harmonics with synthesized two- or three-colour laser fields. Nat. Commun. 5:4003 doi: 10.1038/ncomms5003 (2014).